Time-domain classification of charge-density-wave insulators Distinguishing insulators by the dominant type of interaction is a central problem in condensed matter physics. Basic models include the Bloch-Wilson and the Peierls insulator due to electron–lattice interactions, the Mott and the excitonic insulator caused by electron–electron interactions, and the Anderson insulator arising from electron–impurity interactions. In real materials, however, all the interactions are simultaneously present so that classification is often not straightforward. Here, we show that time- and angle-resolved photoemission spectroscopy can directly measure the melting times of electronic order parameters and thus identify—via systematic temporal discrimination of elementary electronic and structural processes—the dominant interaction. Specifically, we resolve the debates about the nature of two peculiar charge-density-wave states in the family of transition-metal dichalcogenides, and show that Rb intercalated 1 T -TaS 2 is a Peierls insulator and that the ultrafast response of 1 T -TiSe 2 is highly suggestive of an excitonic insulator. Metal-insulator transitions have a prominent role in condensed matter physics, not only as a source of spectacular resistivity changes over many orders of magnitude that may form the basis of electronic devices, but also particularly as a major intellectual challenge driving the development of theoretical and experimental methods [1] , [2] , [3] , [4] , [5] . The active interest in the field is largely due to the fact that one is confronted with a many-body problem. As any metal-insulator transition is driven by a variety of interactions between the many electronic and structural degrees of freedom constituting a solid, the phenomenon represents an excellent test of our understanding of complex systems [4] . In systems dominated by electron–electron and electron–phonon interactions, there are three distinct models of insulators, all connected with the emergence of long-range charge order and a gap in the electronic structure at the Fermi energy E F ( Fig. 1 ) [2] , [5] . The first model is the Mott insulator, resulting from the intra-atomic Coulomb interaction. Mott insulators can arise from metals with a flat band straddling E F . They are characterized by the complete localization of the valence electrons at the atomic sites and by the opening of a density-of-states gap at E F ( Fig. 1a ). The second model is the excitonic insulator, arising from the unscreened electron–hole interaction. An excitonic instability due to the spontaneous formation of excitons can occur in a semimetal with a small overlap or a semiconductor with a small gap and may lead to a charge-density wave (CDW). The CDW phase is accompanied by a small, 'accidental' lattice distortion due to finite electron–phonon coupling, and is stabilized by a gap at E F due to an avoided crossing of the valence and conduction bands ( Fig. 1b ). The third model is the Peierls insulator, resulting from electron–phonon interactions. In a Peierls instability, the formation of a CDW and a periodic lattice distortion go hand in hand. The wavelength and symmetry of the periodic modulations fit to the Fermi surface such that occupied electronic states near E F are lowered and the resulting gain in electronic band energy is larger than the cost in Coulomb and lattice energy ( Fig. 1c ). 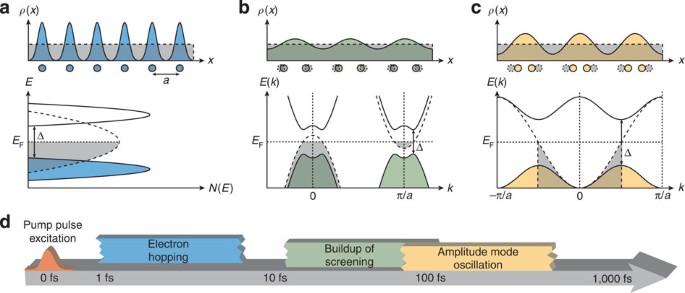Figure 1: Three basic classes of insulators and their characteristic response times. (a) Mott insulator. (b) Excitonic insulator. (c) Peierls insulator. For each case, the characteristic signatures of the insulating state (solid lines, coloured shading) following the transition from a metallic state (dashed lines, grey shading) are illustrated: in real space, the periodic modulation of the valence-electron density and, if applicable, of the atomic positions, and in energy-momentum space, the opening of an energy gap (Δ). (d) Corresponding timescales of the responses to impulsive near-infrared excitation, as derived from the materials investigated in the present work, and their assignment to elementary model-specific processes. Figure 1: Three basic classes of insulators and their characteristic response times. ( a ) Mott insulator. ( b ) Excitonic insulator. ( c ) Peierls insulator. For each case, the characteristic signatures of the insulating state (solid lines, coloured shading) following the transition from a metallic state (dashed lines, grey shading) are illustrated: in real space, the periodic modulation of the valence-electron density and, if applicable, of the atomic positions, and in energy-momentum space, the opening of an energy gap (Δ). ( d ) Corresponding timescales of the responses to impulsive near-infrared excitation, as derived from the materials investigated in the present work, and their assignment to elementary model-specific processes. Full size image Classification according to the above scheme, however, is often not straightforward because in real complex materials, electron–electron and electron–phonon interactions are often simultaneously strong and the dominant interaction is not easily identified. An important part of the problem is that the characteristic signature of the resulting insulating state, the gap in the electronic spectrum as observed in (time-integrated) spectroscopy, may look the same in all the three cases. The central hypothesis of the present work is that complex insulators can be classified more reliably in the time domain—by time- and momentum-resolved pump-probe spectroscopy—on the basis of the gap melting times. The underlying idea is that the length and excitation density dependence of the melting time should directly reflect an elementary interaction-dependent process specific to each class of insulator ( Fig. 1d ). This hypothesis is here tested using a set of transition-metal dichalcogenides, layered materials that continue to provide a fertile field for disentangling the combined effects of electron–phonon and electron–electron interactions, in pristine compounds [6] as well as in intercalation complexes [7] . Two prominent examples are 1 T -TaS 2 and 1 T -TiSe 2 . In these two compounds, the electronic structures [8] , [9] , [10] , [11] , [12] , [13] , [14] , [15] and ultrafast spectral responses [16] , [17] , [18] , [19] indicate the presence of significant electron correlation effects. In both compounds, electron–electron interactions may in fact have an important role in CDW formation [12] , [13] , [14] , [18] , [19] , [20] and in the emergence of superconductivity from CDW states upon intercalation [21] or under pressure [22] , [23] . Systems The momentum-space symmetries of the three arguably most intriguing CDW phases of 1 T -TaS 2 and 1 T -TiSe 2 , are shown in Fig. 2 , together with the unreconstructed schematic Fermi surfaces and the reconstructed band structures as seen by (time-integrated) angle-resolved photoemission spectroscopy (ARPES). 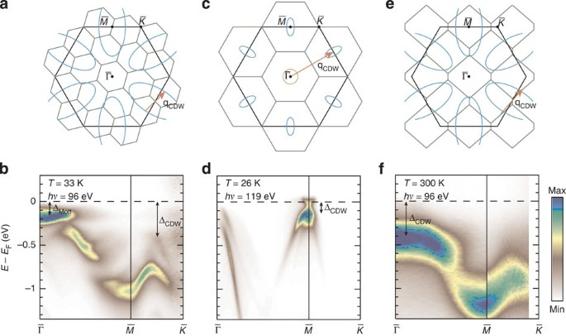Figure 2: Static momentum-space view of three charge-density-wave phases in layered transition-metal dichalcogenides. Reconstructed (green lines) and original (black lines) projected Brillouin zones (top row) and measured band dispersions along thehigh-symmetry path (bottom row) for (a,b) thephase of 1T-TaS2(c,d) thep(2×2×2) phase of 1T-TiSe2and (e,f) thephase of Rb:1T-TaS2. In (a,c,e), unreconstructed schematic Fermi surfaces (circle and ellipses), wavevectors of the CDW (arrows) and high-symmetry points of the original Brillouin zones (dots) are indicated. For illustrative purposes, unreconstructed 1T-TiSe2is assumed to be semimetallic. In (b,d,f), temperatures and photon energies of the ARPES measurements are indicated. Photoemission intensity is represented in a false-colour scale. The arrows mark characteristic energy gaps in the spectra. Figure 2: Static momentum-space view of three charge-density-wave phases in layered transition-metal dichalcogenides. Reconstructed (green lines) and original (black lines) projected Brillouin zones (top row) and measured band dispersions along the high-symmetry path (bottom row) for ( a , b ) the phase of 1 T -TaS 2 ( c , d ) the p (2×2×2) phase of 1 T -TiSe 2 and ( e , f ) the phase of Rb:1 T -TaS 2 . In ( a , c , e ), unreconstructed schematic Fermi surfaces (circle and ellipses), wavevectors of the CDW (arrows) and high-symmetry points of the original Brillouin zones (dots) are indicated. For illustrative purposes, unreconstructed 1 T -TiSe 2 is assumed to be semimetallic. In ( b , d , f ), temperatures and photon energies of the ARPES measurements are indicated. Photoemission intensity is represented in a false-colour scale. The arrows mark characteristic energy gaps in the spectra. Full size image The reconstruction of pristine 1 T -TaS 2 ( Fig. 2a ), which occurs at temperatures below 180–200 K (depending on cooling or heating), is rather well understood as a combined Peierls–Mott insulating phase [8] , [10] , [24] : the strong periodic lattice distortion, which is coupled to the CDW, splits the occupied part of the lowest-lying Ta 5 d band into three subband manifolds so that the uppermost, half-filled manifold becomes susceptible to a Mott-Hubbard-type transition creating a deep pseudogap at E F . The spectroscopic signatures of this scenario are remarkably strong and momentum selective. In the ARPES spectral weight distribution depicted in Fig. 2b , the Mott-Hubbard gap (taken here as the distance between E F and the lower Hubbard band) has a size of about 120 meV and is best visible near the point [8] . The CDW reconstruction, on the other hand, seems most pronounced in the clear subband splittings along , the strong band backfolding along and the large spectral gap of about 400 meV that opens at the edge of the original Brillouin zone (midway between and ). The latter feature may be understood as the projection of the original, nesting-induced gap of the high-temperature incommensurate CDW phase into the low-temperature commensurate phase [15] (as indicated by the nesting vector in Fig. 2a ). Second, there is the conspicuous p (2 × 2 × 2) CDW phase ( Fig. 2c ) of pristine 1 T -TiSe 2 , appearing below 200 K [25] , whose microscopic origin has remained elusive for more than three decades. On the one hand, quantitative microscopic explanations [26] are difficult and deviate too much from experiment [12] , [13] , [14] . On the other hand, qualitative explanations in terms of an electron-lattice instability (variously called Peierls instability, band-type/indirect Jahn-Teller effect or antiferroelectric transition) [12] , [25] , [27] , [28] , [29] , a purely electronic phenomenon (an excitonic insulator instability) [14] , [20] , [30] , or a combination of the two scenarios [13] , [31] are ambiguous as they all seem consistent with subsets of the extensive body of experimental and theoretical results. All proposed models explicitly involve the interaction between the Se 4 p valence band maximum at and the conduction band minimum at , the band extrema that are 'nested' by the wavevector of the CDW and mapped onto each other in the CDW phase ( Fig. 2c ). The spectral weight distribution in Fig. 2d shows that the ensuing direct band repulsion results in a gap of about 100 meV between the lowest-lying Ti 3 d states and the strikingly intense Se 4 p states folded to the original point. The controversy about the CDW mechanism is ultimately about the nature of this p – d interaction, about whether it is predominantly phononic or excitonic. The third peculiar CDW phase occurs in intercalation complexes of 1 T -TaS 2 (ref. 32 ), in particular upon in situ Rb intercalation of pristine 1 T -TaS 2 (Rb:1 T -TaS 2 ) at room temperature [33] , [34] . The phase is characterized by a non-hexagonal . CDW superlattice ( Fig. 2e ) and, in the measured spectral weight distribution, by a surprisingly large energy gap of about 400 meV in the Ta 5 d states at E F around the point ( Fig. 2f ). However, the nature of this gap is presently unclear: while the intercalation-induced change of CDW symmetry clearly points to a Peierls gap, the magnitude and weak momentum dependence of the gap, the absence of Fermi surface nesting ( Fig. 2e ), and the lack of substructure in the band dispersion rather suggest the gap to be of the Mott type [33] , [34] . In summary, the three selected CDW phases confront us with three intriguing variations of the possible interplay of electron–phonon and electron–electron (electron–hole) interactions in the formation of a gapped ground state, in each case raising the intertwined questions about the nature of this ground state and the origin of the transition. In addition, the selection of materials allows for a systematic exploration of these questions because after all the unreconstructed systems exhibit the same basic structure and, despite their distinct band structures, a similar density of states near E F [15] . For pristine 1 T -TaS 2 the question seems indeed settled: the material is a Peierls-Mott insulator, in which the Peierls instability provides a sufficient condition for the Mott transition to occur. But for the other two systems the situation is unclear and the general classification problem reduces to the two specific questions: Is Rb:1 T -TaS 2 a Mott or a Peierls insulator and is 1 T -TiSe 2 a Peierls or an excitonic insulator? Time-resolved ARPES We now set out to answer these questions by time-resolved pump-probe ARPES [16] , [17] , [18] , [19] , [35] , [36] using a high-harmonic-generation source [37] , [38] . The central idea is that the timescale on which electronic order in momentum space melts should provide a strong hint as to its predominant nature or origin. To verify this idea, we will establish a hierarchy of melting times for different types of spectral features in the three systems that shall allow us to identify the dominant interaction behind the gapped phases of Rb:1 T -TaS 2 and 1 T -TiSe 2 , if we use the characteristic momentum-dependent spectral response of 1 T -TaS 2 [16] , [17] , [18] , [39] , [40] as a reference. Specifically, we will compare and contrast the dynamics of the Ta 5 d gap at in Rb:1 T -TaS 2 ( Fig. 2f ) and the folded Se 4 p spectral weight at in 1 T -TiSe 2 ( Fig. 2d ) with the dynamics of the Mott gap at and the Peierls gap near in pristine 1 T -TaS 2 ( Fig. 2b ). In our time-resolved ARPES experiments, to facilitate a systematic comparison and reveal any excitation-density dependence, the four 'spectroscopic order parameters' in the three different materials are quenched under identical excitation conditions for two different excitation densities. All samples are held at an equilibrium temperature of 110 K and are impulsively excited with 30 fs (FWHM), 790 nm near-infrared pulses at constant absorbed energy densities of 300 and 600 Jcm −3 . At these excitation densities, the lattice temperatures in all three systems will transiently increase by 163±21 and 314±41 K, respectively, enough to drive pristine 1 T -TaS 2 and 1 T -TiSe 2 across thermal phase transitions (see Methods ). Yet, the ARPES snapshots in Fig. 3a-d display qualitative electronic structure changes happening within 65–210 fs after excitation, which is much faster than the 0.35–4 ps it takes to transfer the excess energy in the electron system to the phonon bath [16] , [17] , [19] , [39] , [40] , [41] . These changes therefore do not reflect transitions to quasi-equilibrium states at elevated effective temperatures, although the band maps look fairly similar to temperature-dependent equilibrium ARPES data [9] , [12] , [13] , [14] . 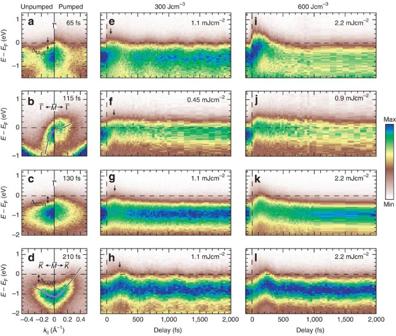Figure 3: Time-resolved momentum-space view of the electronic structure in layered charge-density-wave compounds. (a–d) ARPES snapshots taken before optical pumping and at characteristic pump-probe delays: (a) at thepoint of 1T-TaS2(b) at thepoint of 1T-TiSe2(c) at thepoint of Rb:1T-TaS2and (d) at thepoint of 1T-TaS2(absorbed pump energy density: 300 Jcm−3; equilibrium temperature: 110 K). Solid lines in (b,d) are guides to the eye. Arrows in (a,c,d) mark energy gaps. (e–l) Time-dependent ARPES spectra at selected momenta for absorbed pump energy densities of (e–h) 300 Jcm−3and (i–l) 600 Jcm−3: (e,i) at thepoint of 1T-TaS2, (f,j) at thepoint of 1T-TiSe2, (g,k) at thepoint of Rb:1T-TaS2, and (h,l) near thepoint of 1T-TaS2. The respective absorbed pump fluences are indicated. Arrows in (e–h) mark the pump-probe delays of the data shown in the right panels of (a–d). The momentum intervals over which the energy distribution curves have been integrated are [0,0.1] Å−1in (e–g,i–k) and [0.2, 0.3] Å−1in (h,l). Figure 3: Time-resolved momentum-space view of the electronic structure in layered charge-density-wave compounds. ( a – d ) ARPES snapshots taken before optical pumping and at characteristic pump-probe delays: ( a ) at the point of 1 T -TaS 2 ( b ) at the point of 1 T -TiSe 2 ( c ) at the point of Rb:1 T -TaS 2 and ( d ) at the point of 1 T -TaS 2 (absorbed pump energy density: 300 Jcm −3 ; equilibrium temperature: 110 K). Solid lines in ( b , d ) are guides to the eye. Arrows in ( a , c , d ) mark energy gaps. ( e – l ) Time-dependent ARPES spectra at selected momenta for absorbed pump energy densities of ( e – h ) 300 Jcm −3 and ( i – l ) 600 Jcm −3 : ( e , i ) at the point of 1 T -TaS 2 , ( f , j ) at the point of 1 T -TiSe 2 , ( g , k ) at the point of Rb:1 T -TaS 2 , and ( h , l ) near the point of 1 T -TaS 2 . The respective absorbed pump fluences are indicated. Arrows in ( e – h ) mark the pump-probe delays of the data shown in the right panels of ( a – d ). The momentum intervals over which the energy distribution curves have been integrated are [0,0.1] Å −1 in ( e – g , i – k ) and [0.2, 0.3] Å −1 in ( h , l ). Full size image The most prominent spectral changes are, on the one hand, the (partial) collapses of the various energy gaps at E F in 1 T -TaS 2 ( Fig. 3a,d ) and in Rb:1 T -TaS 2 ( Fig. 3c ), essentially resulting from shifts of the topmost spectral features to higher energies, and, on the other hand, the suppression of the superstructure peak in 1 T -TiSe 2 at the point ( Fig. 3b ), as indicated by the transfer of spectral weight to electron states above E F , the narrowing of the spectrum at , and the apparent switch of the band dispersion from hole-like to electron-like [19] . We also note that despite the poorer energy resolution compared to the synchrotron data of Fig. 2, all four 'spectroscopic order parameters' are clearly resolved in Fig. 2a–d and that the impulsive near-infrared pumping does not degrade the resolution. Figure 3e–l shows the corresponding diverse electronic structure dynamics at selected momenta for the two pump densities used, displaying temporal responses that vary significantly in their rise time, character of the decay and excitation density dependence. The initial closings of the Mott gap and the Peierls gap in the reference compound 1 T -TaS 2 are clearly seen as the fastest and slowest processes, respectively, with rise times of <50 and ~200 fs that seem to be independent of the excitation density ( Fig. 3e,h,i,l ). On longer timescales, the time-resolved ARPES spectra at the corresponding momenta are periodically modulated, as is particularly obvious for the lower excitation density ( Fig. 3e,h ). This oscillatory component in the spectral response is known to reflect the coherent amplitude-mode oscillations of the CDW which in 1 T -TaS 2 couple strongly to the electrons near E F [16] , [18] . At the higher excitation density, these oscillations are strongly damped and become anharmonic ( Fig. 3i,l ) [42] . Figure 3f,j,g,k shows that the melting of the superstructure peak at in 1 T -TiSe 2 and the closing of the energy gap at in Rb:1 T -TaS 2 happen on intermediate timescales and that the oscillations in the spectral responses are completely suppressed, except for a barely visible oscillation of the leading valence-band edge in Rb:1 T -TaS 2 at the lower excitation density ( Figs 3g and 4 ). For 1 T -TiSe 2 , the absence of coherent amplitude-mode oscillations is consistent with time-resolved optical reflectivity results which show that these oscillations are strongly damped at the sample temperature and excitation densities used in our experiments [41] . A distinctive feature of the electronic structure dynamics of 1 T -TiSe 2 is that the melting time of the superstructure peak is dependent on the excitation density, the faster melting occurring at the higher density (see energy range between −0.6 and −0.2 eV between 0 and 100 fs in Fig. 3f,j ) [19] . 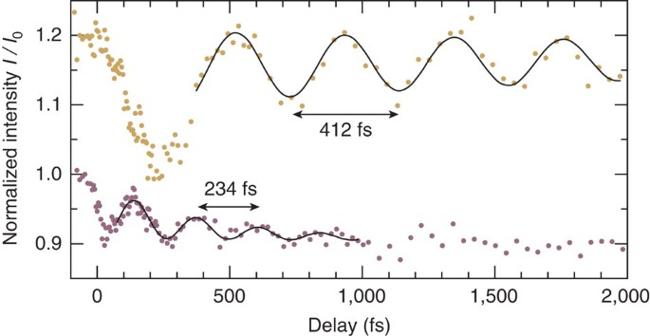Figure 4: Oscillatory spectral responses in 1T-TaS2and Rb:1T-TaS2. Time dependence of the ARPES intensity in selected energy intervals of the transient energy distribution curves shown inFig. 3g,h(absorbed pump energy density: 300 Jcm−3). The experimental data for 1T-TaS2near thepoint (gold dots) and Rb:1T-TaS2at thepoint (violet dots) are compared with fits to a sine function with an exponentially decreasing amplitude (solid lines). The best-fit values for the oscillation period are indicated. Intensities are normalized to the average intensityI0in the delay interval [−500,−50] fs; curves are offset for clarity. The energy intervals over which the intensity has been integrated are [−2,−1] eV for 1T-TaS2and [−1.2,0] eV for Rb:1T-TaS2. Figure 4: Oscillatory spectral responses in 1 T -TaS 2 and Rb:1 T -TaS 2 . Time dependence of the ARPES intensity in selected energy intervals of the transient energy distribution curves shown in Fig. 3g,h (absorbed pump energy density: 300 Jcm −3 ). The experimental data for 1 T -TaS 2 near the point (gold dots) and Rb:1 T -TaS 2 at the point (violet dots) are compared with fits to a sine function with an exponentially decreasing amplitude (solid lines). The best-fit values for the oscillation period are indicated. Intensities are normalized to the average intensity I 0 in the delay interval [−500,−50] fs; curves are offset for clarity. The energy intervals over which the intensity has been integrated are [−2,−1] eV for 1 T -TaS 2 and [−1.2,0] eV for Rb:1 T -TaS 2 . Full size image The oscillatory components in the spectral responses of pristine and Rb intercalated 1 T -TaS 2 are analysed in Fig. 4 by plotting the ARPES intensities within selected energy intervals as a function of the pump-probe delay. The observed period of the amplitude-mode oscillation in pristine 1 T -TaS 2 is τ amp =412±5 fs and agrees reasonably well with the bulk value of about 425 fs measured by time-resolved optical reflectivity at 120 K (ref. 43 ). The difference may be explained by the fact that our ARPES measurements, which employ extreme ultraviolet (XUV) radiation, are highly surface sensitive and probably only probe the stiffer surface amplitude mode [16] . In Rb:1 T -TaS 2 , the amplitude of the oscillation is smaller, the damping stronger and τ amp =234±6 fs shorter by almost a factor of two, all of which strongly indicate that the properties of the collective CDW excitations are significantly modified upon the Rb intercalation-induced transition to the phase. However, what is important for the following quantitative analysis is that the experimentally determined values of τ amp (or some fraction thereof) define an intrinsic timescale for the fastest possible structural response in the two systems [16] , [17] , [35] , [36] , [40] . 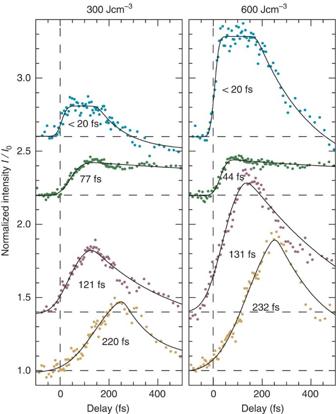Figure 5: Hierachy of melting times of electronic order parameters in layered charge-density-wave compounds. Time dependence of the ARPES intensity in selected energy intervals of the transient energy distribution curves shown inFig. 3e–lfor two absorbed pump energy densities of 300 Jcm−3(left column) and 600 Jcm−3(right column). The experimental data for 1T-TaS2at thepoint (blue dots, first row), 1T-TiSe2at thepoint (green dots, second row), Rb:1T-TaS2at thepoint (violet dots, third row) and 1T-TaS2near thepoint (gold dots, fourth row) are compared with fits to a model function described in the Methods section. The best-fit values for the melting time constants are indicated. Intensities are normalized to the average intensityI0in the delay interval [−500,−50] fs; curves are offset for clarity. Note that for better comparison, the curves for 1T-TiSe2have been inverted (they represent intensity losses in the chosen energy interval, whereas all other curves show intensity increases). The energy intervals over which the intensity has been integrated are [−0.12,0] eV at thepoint of 1T-TaS2, [−1.0,−0.4] eV at thepoint of 1T-TiSe2and [−0.4,0] eV at thepoint of Rb:1T-TaS2and near thepoint of 1T-TaS2. Figure 5 shows characteristic ARPES intensity transients, extracted from the data in Fig. 3e–l , that allow us to quantify how fast the various electronic order parameters are quenched (note that for better comparison the order-parameter transients of 1 T -TiSe 2 have been inverted). These transients also reveal part of the complex relaxation dynamics that will not be further investigated here. The detailed shape of the transients after the initial exponential rise generally depends on several intrinsic and extrinsic factors including the rate of electron-phonon thermalization, the presence and onset of coherent amplitude-mode oscillation, and the nature of the quasi-equilibrium state being reached, as well as the choice of the integration window and normalization procedure. The interplay of these factors can, for example, produce the plateau in the order-parameter transient of 1 T -TaS 2 , to which we do not attribute a specific cause, and the seemingly slower relaxation dynamics of 1 T -TiSe 2 , which does in fact happen on the picosecond timescale [19] . By contrast, because of its ultrashort timescale, the analysis of the melting dynamics is significantly more robust. Figure 5: Hierachy of melting times of electronic order parameters in layered charge-density-wave compounds. Time dependence of the ARPES intensity in selected energy intervals of the transient energy distribution curves shown in Fig. 3e–l for two absorbed pump energy densities of 300 Jcm −3 (left column) and 600 Jcm −3 (right column). The experimental data for 1 T -TaS 2 at the point (blue dots, first row), 1 T -TiSe 2 at the point (green dots, second row), Rb:1 T -TaS 2 at the point (violet dots, third row) and 1 T -TaS 2 near the point (gold dots, fourth row) are compared with fits to a model function described in the Methods section. The best-fit values for the melting time constants are indicated. Intensities are normalized to the average intensity I 0 in the delay interval [−500,−50] fs; curves are offset for clarity. Note that for better comparison, the curves for 1 T -TiSe 2 have been inverted (they represent intensity losses in the chosen energy interval, whereas all other curves show intensity increases). The energy intervals over which the intensity has been integrated are [−0.12,0] eV at the point of 1 T -TaS 2 , [−1.0,−0.4] eV at the point of 1 T -TiSe 2 and [−0.4,0] eV at the point of Rb:1 T -TaS 2 and near the point of 1 T -TaS 2 . Full size image Using a simple phenomenological model function (described in the Methods section), we can establish the envisioned hierarchy of melting time constants and link it to the timescales of elementary electronic and structural processes (as illustrated in Fig. 1d ). The reference timescales are set by pristine 1 T -TaS 2 (top and bottom row of Fig. 5 ). The Mott gap collapses quasi-instantaneously within the duration of the pump pulse (30 fs FWHM), with a time constant of less than 20 fs, in agreement with the results of a recent time-resolved ARPES study [18] . This ultrashort timescale is direct evidence for the electronic origin of the gap; it is consistent with an electronic hopping time , which sets the timescale for the response of the correlated electron system to sudden changes [44] , [45] (here W= 80–400 meV corresponds to the width of the split-off Ta 5 d band that straddles E F [10] , [16] , [11] ). The melting of the Peierls gap, by contrast, takes at least one order of magnitude longer, about 226±38 fs. This value corresponds to half an oscillation cycle of the amplitude mode τ amp /2=206 fs, a connection which is immediately visible in Fig. 3h, l and a clear indication for the structural origin of the gap. The same fingerprint of Peierls physics is seen in the melting of the energy gap in Rb:1 T -TaS 2 , though on a shorter timescale (third row of Fig. 5 ). The melting time constant is 126±20 fs and agrees well with the structural timescale, τ amp /2=117 fs. The suppression of the superstructure peak in 1 T -TiSe 2 , on the other hand, is qualitatively different and cannot be classified as easily (second row of Fig. 5 ). The process is slower than electron hopping ( τ hop <1 fs for W ≳ 1eV (ref. 20 )), but faster than atomic motion ( τ amp /2>160 fs at 110 K (ref. 41 )), and notably in contrast to the other processes, its timescale depends on the excitation energy density and thus on the number of excited carriers [19] . The extracted time constants are 77±9 and 44±14 fs for 300 and 600 Jcm −3 , respectively, and they are in fact in remarkably good agreement with the characteristic times needed for the buildup of screening, 68 and 54 fs, as estimated from the common formula for the plasma frequency [19] , [46] , [47] , [48] , [49] (see Methods ). The sub-100 fs sub-vibrational melting time, its distinct excitation density dependence and the accordance with free carrier screening then all point to a predominantly electronic phenomenon in 1 T -TiSe 2 . The systematic comparison of spectral responses under identical excitation conditions and the direct connection of the observed timescales to elementary processes involving the electrons and the lattice thus lead us to conclude that the puzzling CDW phases of Rb:1 T -TaS 2 and 1 T -TiSe 2 are dominated by electron–phonon interactions and by electron–electron interactions, respectively. In other words, Rb:1 T -TaS 2 is a Peierls insulator, whereas 1 T -TiSe 2 is indeed an excitonic insulator. To further support these claims, we will now briefly discuss our time-resolved ARPES results in the context of some important recent experimental findings on the same systems. The key experimental advance of our study of the reference material 1 T -TaS 2 is to determine the electronic structure dynamics near the edge of the unreconstructed Brillouin zone, specifically in the region of momentum space in which the nesting-induced gap opens up to stabilize the periodic lattice distortion of the high-temperature incommensurate CDW phase ( Fig. 2a,b ). This is the region in which the primary structural component of the CDW in 1 T -TaS 2 can be probed, as confirmed by the vibrational timescale of the spectral response and consistent with the delayed response seen in paradigmatic CDW systems [35] , [50] . In a recent time-resolved ARPES study of 1 T -TaS 2 (ref. 18 ), by contrast, only the region around was probed and, due to the better energy resolution compared with our experiment, a sub-vibrational collapse of the subband splitting at about 250 meV below E F ( Fig. 2b ) was observed. This region of momentum space therefore seems more appropriate to probe the secondary electronic component of the CDW in 1 T -TaS 2 , which, however, may be intertwined with the Mott physics that emerges at the lock-in transition to the low-temperature commensurate CDW phase. The identification of Rb:1 T -TaS 2 as a Peierls insulator rests on the clear spectroscopic fingerprint of lattice dynamics that has been established for the reference 1 T -TaS 2 . The time-resolved ARPES results fully corroborate the conclusions presented in a recent time-integrated ARPES study [34] . Because of the remarkably large and extended energy gap, the Rb:1 T -TaS 2 should in fact be classified as a Peierls insulator in the strong-coupling regime, in which Fermi surface nesting does not have a role anymore [15] , [51] . The time-domain classification of 1 T -TiSe 2 as an excitonic insulator may be more controversial. The argument comprises not only the shortness of the order-parameter melting time but also its distinct fluence dependence [19] and consistency with screening as the essential ingredient of the excitonic insulator instability [1] , [52] , [53] . Although we have previously advanced this argument [19] , the potential uniqueness of the spectral response has remained unclear. It is the context of time-resolved ARPES results obtained from CDW systems of the same family of compounds which now establishes this uniqueness and thus constitutes, in our view, the most conclusive evidence for the existence of the excitonic insulator phase in 1 T -TiSe 2 to date: the ultrafast spectral response of 1 T -TiSe 2 is clearly different from that of the paradigmatic Peierls insulator. This claim does not conflict with the complete phonon softening observed in recent inelastic X-ray scattering measurements [54] because in an excitonic CDW instability the actual soft mode is a mixed exciton-phonon mode so that the electronically driven CDW is always accompanied by a periodic lattice distortion [53] , [55] . Regarding the energy density needed to melt the CDW nonthermally, however, our time-resolved ARPES results are inconsistent with recent time-resolved X-ray diffraction measurements [41] . This is an open issue, but we would argue that for an excitonic insulator, it is more appropriate to monitor the electronic order-parameter dynamics rather than the dynamics of the periodic lattice distortion which may in fact be regarded as an accidental byproduct of the excitonic insulator instability due to finite electron–phonon coupling [55] . Yet, we also emphasise that the melting dynamics we focus on here provides a handle only on the predominant character of the phase being destroyed, but not on the origin of the transition to this phase. Electron–phonon coupling may therefore still be an important trigger for CDW formation in 1 T -TiSe 2 . On a general level, our results then demonstrate that different types of long-range electronic order are indeed quenched on different characteristic timescales and that notably a CDW, being generally composed of a lattice charge density and of an electronic charge density [52] , can melt either on a structural timescale, as in the Peierls insulator Rb:1 T -TaS 2 , or on an electronic timescale, as in the excitonic insulator 1 T -TiSe 2 , or on both timescales, as in the Peierls-Mott insulator 1 T -TaS 2 (ref. 18 ), depending on which density component or underlying interaction is the dominant one (at the probed momentum). The observed hierarchy of melting times ultimately seems to reflect three different non-thermal destruction mechanisms following photoexcitation ( Fig. 1d ): the Mott insulator collapses due to an ultrafast non-equilibrium rearrangement of the electronic states taking place on the elementary timescale of electron hopping [44] , the excitonic insulator breaks down because the Coulomb attraction causing electrons and holes to form excitons is screened by the added free carriers as soon as screening has built up on the timescale of the inverse plasma frequency [19] , and the Peierls insulator melts via a displacive excitation of coherent atomic motions resulting in a suppressed periodic lattice distortion within about half an oscillation of the amplitude mode [40] . In conclusion, the direct, momentum-selective and systematic observation of electronic order parameter dynamics on the relevant timescales, as demonstrated here using time-resolved ARPES, offers a powerful and intuitive approach to assess the relative contributions of electron–electron and electron–phonon interactions to electronic order in momentum space: the very timescale on which the dynamics takes place, together with its excitation density dependence, uncovers the dominant interaction. The approach may help not only to capture the intermediate grades between pure Mott, Peierls and excitonic insulators but also to distinguish different types of gaps in, for example, unconventional superconductors. Sample preparation 1 T -TaS 2 and 1 T -TiSe 2 single crystals were grown from high purity elements by chemical vapour transport using iodine as transport agent. Sample quality was checked by electronic transport measurements. In the photoemission experiments, all samples were cleaved under ultrahigh vacuum conditions at room temperature. The Rb:1 T -TaS 2 samples were prepared in situ by depositing Rb for 300 s on freshly cleaved 1 T -TaS 2 surfaces at room temperature (using a SAES getters dispenser operating at a current of 6 A and a working distance of about 3 cm). Photoemission measurements Time-integrated ARPES measurements were performed at beamline 7.0.1 of the Advanced Light Source at Berkeley employing a Scienta R4000 spectrometer. Typical effective energy and angle resolutions were 90 meV and 0.2°, respectively. The femtosecond time-resolved ARPES experiments were done at the University of Kiel using a SPECS Phoibos 150 analyser. Here, the total energy resolution was 400 meV, mainly governed by the spectral broadening of the femtosecond XUV pulses, and the angle resolution was estimated to be 1.5°. Before each measurement run, the sample orientation and electronic gap sizes were checked by time-integrated ARPES using a He discharge lamp ( hv =21.22 eV). The equilibrium sample temperature was 110 K for all reported time-resolved ARPES data. The basic light source used for pump-probe photoemission was a 3-kHz Ti:sapphire amplifier system (KMLabs Dragon pumped by a Spectra Physics Empower 30) delivering near-infrared pulses at 790 nm wavelength, 1.2 mJ pulse energy and 30 fs (FWHM) pulse duration (representing the major contribution to the effective time resolution of the experiment). For photoemission, 90% of the pulse energy was used to generate high harmonic femtosecond XUV pulses in an argon-filled hollow-fibre waveguide (KMLabs XUUS). A pair of multilayer mirrors (with a total reflectivity of 13%) selected the 27th harmonic ( hv =43 eV) out of the harmonic spectrum and focused it onto the sample mounted in the ultrahigh vacuum system. From infrared-XUV cross-correlation measurements, the pulse duration of the XUV probe pulses was estimated to be shorter than 10 fs. The remaining 10% of the amplifier output were available for photoexcitation of the samples. The s -polarized pump pulses impinged on the sample under 45°, except for measurements around the point of 1 T -TaS 2 for which the incidence angle was about 25° relative to the surface normal. For pristine 1 T -TaS 2 and 1 T -TiSe 2 , the absorbed energy densities and corresponding temperature increases in the excited sample volumes were determined from the measured incident pump fluences using reflection coefficients of 0.41 (ref. 56 ) and 0.65 (ref. 57 ), penetration depths of 36 (ref. 56 ) and 15 nm (ref. 57 ), specific heat β values of 12.6 (ref. 58 ) and 9.45 Jm −3 K −4 (ref. 59 ), and Debye temperatures of 237 (ref. 58 ) and 251 K (ref. 59 ), respectively. In the case of Rb:1 T -TaS 2 , we assumed that the system can be reasonably described by the optical and specific heat parameters of pure 1 T -TaS 2 . Data analysis The temporal evolutions of the ARPES intensities in the energy windows of interest were fitted with a model function composed of the Gaussian error function to capture the fast initial collapse and a single exponential to model the slower relaxation dynamics. The finite time resolution of the experiment was modelled by a convolution with a Gaussian of 32 fs FWHM. The stated melting times correspond to the FWHM of the derivative of the Gaussian error function. The fluence dependent screening times in 1 T -TiSe 2 were estimated from the common formula for the plasma frequency, using a relative electric constant of ε γ =19 (ref. 60 ), an effective isotropic electron mass of (ref. 13 ), a free carrier density of n 0 =0.1 × 10 19 cm −3 (ref. 60 ), an assumed quantum efficiency (QE) of 0.1 and a photon density n derived from the absorbed energy density ( ε 0 : electric constant; e 0 : elementary charge; m e : electron mass). How to cite this article : Hellmann, S. et al . Time-domain classification of charge-density-wave insulators. Nat. Comm. 3:1069 doi: 10.1038/ncomms2078 (2012).